Unraveling quantum pathways using optical 3D Fourier-transform spectroscopy Predicting and controlling quantum mechanical phenomena require knowledge of the system Hamiltonian. A detailed understanding of the quantum pathways used to construct the Hamiltonian is essential for deterministic control and improved performance of coherent control schemes. In complex systems, parameters characterizing the pathways, especially those associated with inter-particle interactions and coupling to the environment, can only be identified experimentally. Quantitative insight can be obtained provided the quantum pathways are isolated and independently analysed. Here we demonstrate this possibility in an atomic vapour using optical three-dimensional Fourier-transform spectroscopy. By unfolding the system’s nonlinear response onto three frequency dimensions, three-dimensional spectra unambiguously reveal transition energies, relaxation rates and dipole moments of each pathway. The results demonstrate the unique capacity of this technique as a powerful tool for resolving the complex nature of quantum systems. This experiment is a critical step in the pursuit of complete experimental characterization of a system’s Hamiltonian. Quantitative knowledge of a system’s Hamiltonian can enable quantitative prediction and control of quantum mechanical systems. A quintessential example is coherent control of quantum phenomena [1] , [2] . Besides the original goal of controlling chemical reactions [3] , [4] , [5] , the applications of coherent control have been extended to a variety of quantum phenomena in different media. For example, experiments have demonstrated control of two-photon transitions in atoms [6] , the shape of an atomic electron’s wavefunction [7] , high-harmonic generation of soft X-rays [8] , energy flow in light-harvesting complexes [9] and coherent processes in bulk semiconductors [10] , quantum wells [11] and dots [12] . The primary principle for coherent control is the manipulation of constructive and destructive interference of quantum pathways between the initial and targeted states [1] , [2] . A remarkable advance toward achieving coherent control is the closed-loop control technique [13] , where an algorithm iteratively learns the pathway information by trial experiments and suggests the next control design until it converges on a targeted state. The technique can, in principle, work without any knowledge of the system, yet the performance of the algorithm strongly depends on suitable initial conditions and proper parameterization [14] , [15] . Except for the simplest cases, the initial and target states are connected by many quantum pathways. Consequently, control is more easily achieved provided sufficient details about each contributing pathway are known. A priori knowledge of the parameters that characterize these pathways—including transition energies, relaxation rates and transition dipole moments—can provide guidance for designing an efficient learning algorithm and satisfactory initial conditions. In general, these parameters are elements of the unperturbed system Hamiltonian, H 0 , and the light-matter interaction Hamiltonian, H I . Using the density matrix ρ , the system dynamics are governed by the equation of motion [16] where H = H 0 + H I , [ H , ρ ]= Hρ − ρH and { Γ , ρ }= Γ ρ + ρ Γ . The matrix elements of H can be written as and H I, ij =− μ ij E ( t ) ( H I, ij =0 for i = j ), where is the energy of state | i ›, E ( t ) is the electric field, μ ij is the dipole moment of the transition between states | i › and | j ›, and δ ij is the Kronecker delta function. The relaxation operator Γ has matrix elements Γ ij =(1/2)( γ i + γ j ), where γ i and γ j are the population decay rates. In general, coherences (off-diagonal density matrix elements) can decay due to pure dephasing processes, such as elastic collisions, in addition to population decay. Pure dephasing cannot be included in equation (1) as it is written. To include pure dephasing, the modified equations of motion for the density matrix elements [16] , must be used, where Γ has been redefined to have elements , and is the pure coherence dephasing rate for i = j ). In the present context, the full Hamiltonian includes both H and Γ , which together determine the time evolution of the density matrix. In principle, the Hamiltonian can be calculated ab initio for a simple system, but it is not practical to calculate the Hamiltonian of a complex system, especially taking into account factors such as inter-particle interactions, incoherent processes and environmental fluctuations. Therefore, components of the Hamiltonian need to be measured in order to correctly include these factors. For example, experimental identification of the potential surface in molecular systems has been approached using inversion procedures, such as the traditional Rydberg–Klein–Rees method [17] , [18] , [19] and optimal identification by closed-loop laser control [20] . However, the inversion methods do not reveal complete system information. In the case of coherent control, it is important to know the parameters characterizing the relevant quantum pathways and relaxation rates [21] . The greatest challenge is how to completely isolate each single pathway so that the information can be unambiguously identified for each particular process. Here, we demonstrate that each pathway can be separated and independently studied using optical three-dimensional Fourier-transform (3DFT) spectroscopy. As a model system, we have experimentally obtained a 3DFT spectrum of a potassium vapour. Within the spectral region covered by our laser, the 3DFT spectrum contains the full third-order coherent response of the vapour, and the spectral contributions from different quantum pathways are unambiguously isolated. Therefore, elements of each quantum pathway, including the transition energies, dipole moments and relaxation rates, can be determined from the spectrum. These measurements provide the necessary information required for a control scheme that uses the same bandwidth pulses and is based on the third-order optical response. In general, the Fourier-transform spectrum needs to have dimensionality that matches the maximum-order nonlinearity used in the control scheme and it needs to be taken with a bandwidth equal to or greater than that to be used for control. Optical 3DFT spectroscopy Optical 3DFT spectroscopy is an extension of optical two-dimensional Fourier-transform (2DFT) spectroscopy, which is itself a powerful tool for studying the coupling and dynamics in complex systems such as photosynthetic proteins [22] , semiconductor quantum wells [23] and quantum dots [24] , [25] . In contrast to one-dimensional spectroscopy, 2DFT spectroscopy spreads a congested spectrum onto a two-dimensional plane and can partially disentangle quantum pathways [26] . 2DFT methods were originally developed in NMR [26] , where it was also found that increasing the dimensionality was beneficial [27] . 2DFT spectroscopy can separate homogeneous and inhomogeneous linewidths by lineshape analysis [28] to give insight into relaxation dynamics. However, 2DFT spectra cannot completely separate quantum pathways and thus do not fully reveal the system’s optical response. In a three-pulse experiment, a 2DFT spectrum has two frequency dimensions corresponding to two time delays, while the third delay is fixed. Information about correlations between coherences associated with this fixed delay is therefore lost and the nonlinear response is not fully unfolded. By taking a series of 2DFT spectra as a function of the third delay, it is possible to observe specific coherences by plotting off-diagonal peak amplitudes as a function of this delay [29] , [30] , [31] ; however, interpreting the dynamics is difficult because absolute frequency information is lost and in many instances multiple contributions to the signal are not fully disentangled. It has been shown [32] that these experimental limitations can be overcome using 3DFT spectroscopy, in which the quantum pathways are further isolated. To completely isolate quantum pathways and obtain the system’s full optical response, we construct 3DFT spectra in three frequency dimensions corresponding to three time delays. Unlike other 3DFT spectroscopy experiments with the objectives of studying fifth-order susceptibility [33] , [34] , [35] , [36] or two-quantum excitation [32] , the aim of our experiment is to extract complete information about the system’s third-order optical response by isolating individual quantum pathways. To isolate individual pathways, the dimensionality of the spectrum must match the order of the nonlinear susceptibility; thus, a 3DFT spectrum based on the fifth-order response cannot extract full information about either the third-order or fifth-order response. 3DFT spectra are generated from a transient four-wave mixing (TFWM) signal, as described in Methods . As shown in Fig. 1a , we denote the time delay between the first and second pulses as τ , between the second and third pulses as T and the emission time as t . The TFWM signal is recorded in the frequency domain while scanning one or two time delays. Multi-dimensional spectra are generated by Fourier transforming the signal with respect to the time delays. A rephasing (non-rephasing) 2DFT spectrum S 1 ( ω τ , T , ω t ) ( S 2 ( ω τ , T , ω t )) is obtained by scanning τ if the conjugated pulse A * arrives first (second). Likewise, scanning T generates a zero-quantum spectrum S 1 ( τ , ω T , ω t ), which can isolate non-radiative zero-quantum coherences [37] . In the present experiment, both τ and T are scanned to construct a 3DFT spectrum S ( ω τ , ω T , ω t ) in three frequency dimensions. Compared to analysing a sequence of 2DFT amplitude spectra taken as a function of T ( [29] , [30] , [31] ), a 3DFT spectrum does a better job of disentangling congested 2D spectra because it identifies zero-quantum coherence frequencies, not just interferences between pathways that give rise to quantum beats, and it correlates frequencies in all three dimensions. 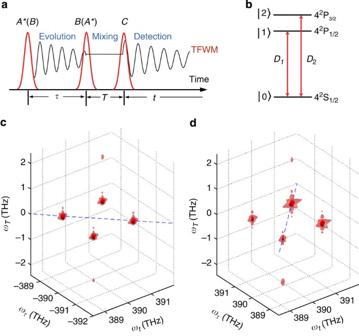Figure 1: 3DFT spectra of a potassium vapour. (a) Time ordering of the three pulses. A rephasing (non-rephasing) spectrum is obtained with the conjugated pulseA* arriving first (second). (b) Relevant energy levels of a potassium atom. (c) Experimental rephasing 3DFT spectrum obtained with pulseA* arriving first. (d) Experimental non-rephasing 3DFT spectrum obtained with pulseA* arriving second. Incanddthe solid red isosurface represents a higher amplitude than the semi-transparent red surface. Blue dashed lines are diagonal lines (ωt=|ωτ|,ωT=0). Figure 1: 3DFT spectra of a potassium vapour. ( a ) Time ordering of the three pulses. A rephasing (non-rephasing) spectrum is obtained with the conjugated pulse A * arriving first (second). ( b ) Relevant energy levels of a potassium atom. ( c ) Experimental rephasing 3DFT spectrum obtained with pulse A * arriving first. ( d ) Experimental non-rephasing 3DFT spectrum obtained with pulse A * arriving second. In c and d the solid red isosurface represents a higher amplitude than the semi-transparent red surface. Blue dashed lines are diagonal lines ( ω t =| ω τ |, ω T =0). Full size image We choose potassium (K) vapour as an illustrative example of how to obtain 3DFT spectra and isolate and characterize individual quantum pathways; however, our approach is applicable to general systems. The D -line transitions between the ground state |0›=|4 2 S 1/2 › and two fine-split states |1›=|4 2 P 1/2 › and |2›=|4 2 P 3/2 › of a K atom form a three-level system ( Fig. 1b ), which is appropriately simple and well characterized [38] to interpret and verify the results and yet sufficiently complex to require the unique capabilities of 3DFT spectroscopy. The D -line transitions are broadened by an argon buffer gas such that the hyperfine and Zeeman sublevels are not resolvable or relevant in our experiments. We have verified that the signal is due to the third-order optical response by measuring the strength of the signal intensity as a function of excitation power and observing a cubic dependence. Typical amplitude 3DFT spectra of K vapour are shown in Fig. 1c . An animation with different viewing angles is available in Supplementary Movie 1 . As a three-dimensional analogue of 2D-contour lines, isosurfaces are plotted to visualize the spectra. The solid red isosurface represents a higher amplitude than the semi-transparent red isosurface. The spectra reveal different quantum pathways that may interfere in the absence of the strict time ordering. The horizontal axes are the absorption ( ω τ ) and emission ( ω t ) frequencies. The vertical axis is the mixing frequency ( ω T ) associated with the zero-quantum coherence between states |1› and |2›. Compared with a 2DFT spectrum, the 3DFT spectrum further unfolds the nonlinear optical response along a third dimension. The contributions from the zero-quantum coherences are isolated from the off-diagonal peaks (rephasing) or the diagonal peaks (non-rephasing) on the ω T =0 plane. Unraveling quantum pathways Unlike one- or two-dimensional spectra, a 3DFT spectrum reveals complete information of the system’s third-order optical response. Various 2DFT spectra can be retrieved by projecting a 3DFT spectrum onto a two-dimensional plane according to the projection-slice theorem of Fourier transforms [26] . For instance, as shown in Fig. 2a and Supplementary Movie 1 , the projection of the rephasing 3DFT spectrum onto the bottom plane ( ω τ , ω t ) is the rephasing 2DFT spectrum at T =0. We can also retrieve the rephasing 2DFT spectrum at any given T using the Fourier shift theorem [26] . Similarly, the zero-quantum 2DFT spectrum at any given τ can be obtained by projecting the 3DFT spectrum onto the left back plane ( ω t , ω T ) with an appropriate phase shift [37] . The projections on the bottom and left back planes are plotted in Fig. 2b . These projections are the spectra that can be acquired by 2DFT spectroscopy; however, the projection onto the right back plane ( ω τ , ω T ) is a unique two-dimensional spectrum that is not accessible by conventional 2DFT techniques based on spectral interferometry. Shown in Fig. 2d , this spectrum is a function of absorption frequency ω τ and mixing frequency ω T , and independent of the emission frequency. Furthermore, this spectrum is not simply time integrated, but corresponds to an instantaneous emission time. This projection on the right back plane can reveal the temporal dynamics of the emission signal in terms of the absorption and mixing frequencies. 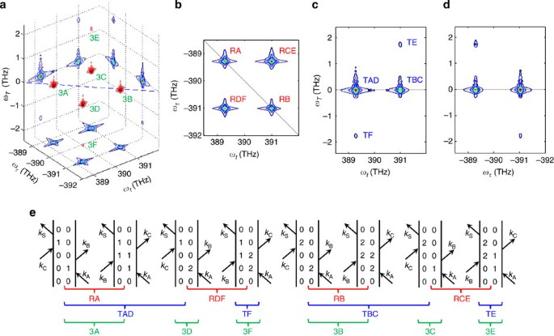Figure 2: Projections and quantum pathways in the 3DFT spectrum. (a) Experimental rephasing 3DFT spectrum fromFigure 1cwith two-dimensional projections on three planes. (b) Projection on the bottom plane, equivalent to a rephasing 2DFT spectrum atT=0. (c) Projection on the left back plane, equivalent to a zero-quantum 2DFT spectrum. (d) Projection on the right back plane, not accessible by conventional 2DFT spectroscopy. (e) Double-sided Feynman diagrams representing all quantum pathways in the system and the corresponding peaks in the spectra. Overlapping pathways in 2DFT spectra are isolated in the 3DFT spectrum. Figure 2: Projections and quantum pathways in the 3DFT spectrum. ( a ) Experimental rephasing 3DFT spectrum from Figure 1c with two-dimensional projections on three planes. ( b ) Projection on the bottom plane, equivalent to a rephasing 2DFT spectrum at T =0. ( c ) Projection on the left back plane, equivalent to a zero-quantum 2DFT spectrum. ( d ) Projection on the right back plane, not accessible by conventional 2DFT spectroscopy. ( e ) Double-sided Feynman diagrams representing all quantum pathways in the system and the corresponding peaks in the spectra. Overlapping pathways in 2DFT spectra are isolated in the 3DFT spectrum. Full size image The most important advantage of 3DFT spectroscopy is the ability to isolate quantum pathways. For the rephasing 3DFT spectrum in Fig. 2a , the contributions from different pathways are isolated in six different peaks labelled 3A–F. However, the 2D spectra ( Fig. 2b–d ) have peaks consisting of the combinations of two 3DFT peaks. More specifically, for the pulse time ordering and the phase-matching condition for the rephasing spectrum, eight different quantum pathways exist that can be represented by the double-sided Feynman diagrams in Fig. 2e . In the traditional rephasing 2DFT spectrum ( Fig. 2b ), each peak (labelled RA, RB, RCE and RDF) has contributions from two different pathways. The off-diagonal peak RCE (RDF) is the projection of two 3DFT peaks 3C and 3E (3D and 3F). The zero-quantum coherence terms can be isolated in the zero-quantum spectrum ( Fig. 2c ) as peaks TE and TF. But the diagonal and off-diagonal 3DFT peaks 3A and 3D (3B and 3C) are combined into the peak TAD (TBC). As illustrated in Fig. 2e , the quantum pathways are most isolated in the 3DFT spectrum where each of the four peaks represents a single pathway. The remaining two peaks 3A and 3B include two pathways each, which describe equivalent processes in the case of a closed system. Therefore, the information on a particular physical process can be unambiguously determined by analysing a single 3DFT spectral peak. For instance, the lineshape and two-dimensional projections of peak 3E can be isolated and analysed ( Fig. 3a ) independently of other peaks. 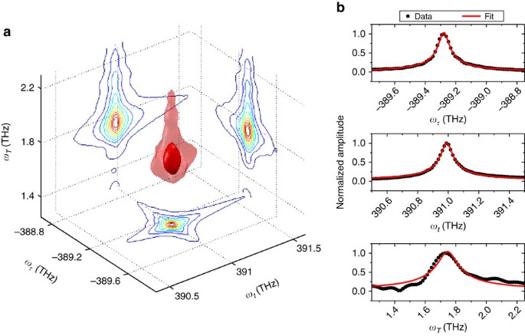Figure 3: Lineshape analysis of a single peak. (a) A single 3DFT spectral peak 3E with projections on three planes. The peak represents a single quantum pathway. The dynamics of the associated process can be understood by analysing lineshape and projections. (b) Profiles of peak 3E along three frequency directions. Dotted lines are data and red lines are fits to a square root of Lorentzian function. Linewidths of the profiles determine the relaxation rates. Figure 3: Lineshape analysis of a single peak. ( a ) A single 3DFT spectral peak 3E with projections on three planes. The peak represents a single quantum pathway. The dynamics of the associated process can be understood by analysing lineshape and projections. ( b ) Profiles of peak 3E along three frequency directions. Dotted lines are data and red lines are fits to a square root of Lorentzian function. Linewidths of the profiles determine the relaxation rates. Full size image Characterizing quantum pathways The 3DFT spectrum provides a complete energy-level scheme rather than just possible transitions that can be inferred from a one-dimensional spectrum. For instance, while an absorption spectrum containing two peaks identifies two transitions, the nature of those transitions is unknown. The energy-level scheme could be a three-level V scheme with two excited states, two independent species of two-level systems, or two two-level systems coupled via incoherent relaxation processes. This uncertainty is absent in a 3DFT spectrum, because these three schemes display different 3D spectral patterns, which are presented in Supplementary Fig. S1 . The spectra observed from K vapour matches the three-level V scheme with two excited states. With the energy level scheme identified, the parameters needed to fully characterize each individual pathway—the transition energy, dipole moment and relaxation rate—can be extracted by analysing an individual peak. For example, solving equation (2) for the pathway associated with peak 3E, the corresponding TFWM signal in the time domain is where N is the atomic density, E A,B,C are the electric field amplitudes of the pulses, ω ij = ω i − ω j , and Θ’s are unit step functions. Fourier transforming the signal into the frequency domain gives the amplitude of peak 3E as Using the notation of the matrix elements of H 0 , H I and Γ defined in equation (2), equation (4) can be rewritten as This equation shows the lineshape profile of peak 3E, which is the square root of a Lorentzian along each frequency axis. The linewidths can be used to extract the elements of Γ , the peak position identifies the elements of H 0 , and the peak amplitude determines the elements of H I . The same analysis is applied to other peaks such that matrices H 0 , H I and Γ can be constructed. We use peaks 3A and 3B to determine two transition frequencies and two dipole moments for the three-level V scheme. The transition frequencies can be identified from the peak positions of 389.3±0.05 and 391.0±0.05 THz. The dipole moments can be determined from the peak strength. The amplitudes of peaks 3A and 3B are related to the dipole moments by and , respectively. Comparing the amplitudes normalized to the laser spectrum provides the relative strength of the dipole moments. The amplitudes of peaks 3A and 3B show μ 02 ≈1.4 μ 01 . Knowing the relative strength is useful for determining the dipole moments that are not accessible by linear spectroscopy (such as for the upper transition in a ladder scheme). The absolute dipole moments can be determined from the atomic density and by measuring the power in the incident beams and the signal beam. In our experiment, the measured dipole moments are μ 01 ≈(1.8±0.83) × 10 −29 C·m and μ 02 ≈(2.5±1.3) × 10 −29 C·m ( Methods ). The relaxation rates are crucial characteristics of the quantum dynamics of a system, and this pathway-dependent information is important for designing coherent control strategies. However, of the parameters required to characterize the quantum pathways, the relaxation rates are the most difficult to determine because the population decay and coherence dephasing in a complex system are affected by many factors. Inter-particle interactions, such as many-body effects, and coupling to the laboratory environment can substantially change the system dynamics. Moreover, isolating the relaxation rates associated with different processes is often difficult. For instance, homogeneous relaxation can be masked by inhomogeneous broadening. Lineshape analysis of multi-dimensional spectral peaks overcomes these difficulties and reveals the relaxation dynamics. For example, a dispersive lineshape in the real part of a 2DFT spectrum is a signature of the many-body interactions between excitons in semiconductors [39] . Homogeneous and inhomogeneous linewidths can also be separated in a 2DFT spectrum of systems with arbitrary inhomogeneity [28] . In a 3DFT spectrum, the pathways are well isolated so that the associated relaxation processes can be identified by analysing the lineshape of the corresponding peak. The lineshape information can be useful for studying many-body physics [40] , [41] . Retrieval of the relaxation rates is demonstrated using lineshape analysis for a single peak 3E ( Fig. 2 ). Peak 3E represents a single pathway involving the zero-quantum coherence between |2› and |1›, which is affected by three relaxation rates: Γ 10 , Γ 20 and Γ 21 . As shown in equation (4), the relaxation rates are isolated in three frequency axes and the profile along each direction is the square root of a Lorentzian. The peak profiles across the peak centre along the three frequency axes are plotted in Fig. 3b . Fits to the square root of a Lorentzian function yield relaxation rates of Γ 10 =34.2±0.7 GHz, Γ 20 =37.5±0.9 GHz and Γ 21 =64.5±7.3 GHz, where the uncertainties are estimated from the least-squares fitting ( Methods ). Comparison of these values yields information about correlation of the fluctuations that cause dephasing. Similar analysis can be performed on peaks 3A and 3B to retrieve relaxation rates Γ 11 =91.5±3.5 GHz and Γ 22 =93.5±5.7 GHz. If the system is inhomogeneously broadened, the homogeneous and inhomogeneous linewidths in each peak can be separated [28] . More complex relaxation processes, for example, non-Markovian, will be evident as non-Lorentzian lines. Analysis of peak 3E demonstrates the unique capability of 3DFT spectroscopy to isolate transitions that are overlapping in 2DFT spectra. This ability is a very important distinction from simply tracking the amplitude of a single point on a series of 2DFT spectra taken at different waiting times [29] , [30] , [31] . In many systems, the dephasing rates Γ 10 and Γ 20 are for optical transitions between potential energy surfaces (in molecules) or bands (in solids). However, Γ 21 will be the dephasing rate between vibrational levels for one potential surface or for intraband transitions, and thus is likely to be much slower as the fluctuations are often correlated. If this is the case, then transitions that are strongly overlapped in the ω t and ω τ dimensions may be well resolved in the ω T dimension. This resolution allows Γ 10 and Γ 20 to be accurately determined from the 3D spectrum, whereas they cannot be from a linear or 2DFT spectrum. This point is illustrated and discussed in Supplementary Fig. S2 . This analysis is repeated for each quantum pathway to determine the transition energies, dipole moments and relaxation rates so that all matrix elements of H 0 , H I and Γ can be identified as shown in Tables 1 , 2 , 3 . We have included uncertainty estimates for completeness; however, we note that the uncertainties in the elements of H I are dominated by uncertainties in the atomic density and laser parameters. These uncertainties would also be present in a coherent control experiment; however, the effects of the uncertainties can be eliminated by performing 3DFT spectroscopy in situ . The values we obtain for H 0 and H I are different from literature values by less than our estimated uncertainty. In addition, the uncertainties in the dipole moments (numeric values in H I,01 and H I,02 ) are correlated, as we can determine the ratio between them to within a few per cent. Table 1 Matrix elements of H 0 . Full size table Table 2 Matrix elements of H I . Full size table Table 3 Matrix elements of Γ . Full size table We have chosen to demonstrate the capabilities of 3DFT spectroscopy for isolating quantum pathways on a relatively simple system, namely one with a single ground state and two excited states. The method will work even if more than two excited states exist, although less sophisticated methods will not work even for the system we use. For a system with additional manifolds of excited states, with each manifold connected by a dipole-allowed transition (often known as a ‘ladder’-type system), our method can still fully determine the third-order optical response, which is sufficient for designing a coherent control scheme that does not access higher-order contributions to the optical response, although it cannot fully determine every element of the Hamiltonian. To fully determine the Hamiltonian for such a system, an N -dimensional spectrum must be measured, where the number of manifolds m is less than N . 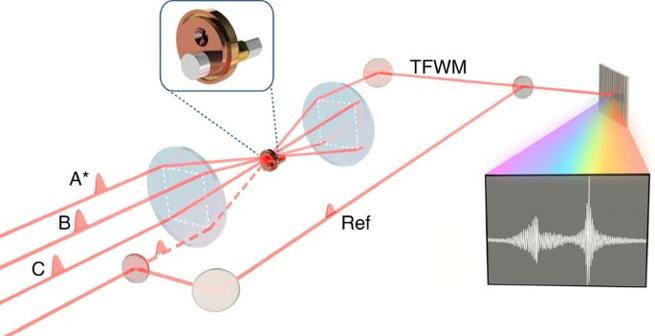Figure 4: TFWM experiment with four beams in the box geometry. Three pulses are incident on the sample to generate a TFWM signal, which is later combined with the reference (Ref) beam for spectral interferometry. The dashed line shows the tracer beam, which is blocked during acquisition of a 3DFT spectrum, but is used to calibrate the phase of the reference. The inset shows the titanium vapour cell. This comparison of techniques and systems is summarized in Table 4 , which is discussed in more detail in the Supplementary Discussion . To demonstrate that we can determine the full third-order nonlinear optical response, even for a ladder system, we have also measured the 3DFT spectrum of a rubidium vapour, where the 5S, 5P and 5D states form a ladder-type configuration. These results are presented in the Supplementary Discussion . Table 4 Capabilities of different methods for determining Hamiltonian. Full size table We have implemented optical 3DFT spectroscopy of atomic vapours. 3DFT spectra contain complete information of the system’s third-order optical response. From a 3DFT spectrum, various 2DFT spectra can be retrieved, including those that are not accessible by conventional 2DFT spectroscopy. The spectral contributions from different interfering quantum pathways are unambiguously isolated. Therefore, each parameter characterizing each quantum pathway, including the transition energies, dipole moments and relaxation rates, can be determined from 3D spectra, to the accuracy permitted by the fact that the optical Bloch equations are themselves an approximation. For a system with a higher-dimensional Hamiltonian, that is, additional levels, more peaks will be present in the 3DFT spectrum; however, it is still sufficient to characterize the quantum pathways as long as levels are in a single manifold and the peaks are resolvable. Applying this technique to other samples, such as semiconductors and molecules, requires proper wavelength and bandwidth of the excitation laser. Thus, optical 3DFT spectroscopy opens an avenue to fully characterize the Hamiltonian of complex systems, which is useful for achieving coherent control of quantum phenomena. Moreover, the ability to extract dynamics of isolated processes can potentially provide insight into the inter-particle interactions in various media. Experimental setup 3DFT spectra are generated from a TFWM signal. As shown in the schematic in Fig. 4 , four phase-stabilized pulses in the box geometry [42] are used for the experiment. Three pulses with wavevectors k A , k B and k C are incident on the sample and generate a TFWM signal in the direction k s =− k A + k B + k C at the fourth corner of the box. The fourth ‘reference’ pulse is routed around the sample and combined with the signal for spectral interferometry. A 3DFT spectrum is generated from a series of interferograms while scanning τ and T . The data acquisition time of each 3DFT spectrum in our experiment is about 25 h, which requires good stability of the setup. The data acquisition time can be substantially reduced by incorporating single-shot 2DFT spectroscopy [43] . Figure 4: TFWM experiment with four beams in the box geometry. Three pulses are incident on the sample to generate a TFWM signal, which is later combined with the reference (Ref) beam for spectral interferometry. The dashed line shows the tracer beam, which is blocked during acquisition of a 3DFT spectrum, but is used to calibrate the phase of the reference. The inset shows the titanium vapour cell. Full size image The K vapour is contained in a titanium cell (inset in Fig. 4 ) with a 1,550-Torr argon buffer gas. The cell has two sapphire windows, between which an ~20 μm layer of K vapour is contained. The atomic density can be adjusted by changing the cell temperature. The layer of K vapour is thin enough such that, at a relatively high atomic density, the absorbance is smaller than one ( αL <1) to eliminate field propagation effects. Uncertainty estimation The uncertainties in relaxation matrix elements ( Γ ij ) are calculated in the least-squares fitting process [44] , which is done with the Nonlinear Curve Fit function in OriginPro 8.6. (Mention of commercial products is for information only; it does not imply NIST recommendation or endorsement, nor does it imply that the products mentioned are necessarily the best available for the purpose.) Take Γ 10 as an example, it is extracted from the slice along the ω τ direction in peak 3E by fitting the data to the function where x i = ω τ is the variable and is the parameter vector. During the Levenberg–Marquardt iteration [44] of the fitting process, the Jacobian matrix J is Then the variance–covariance matrix C for parameters is where s 2 is the mean residual variance. The error of each fitting parameter is the square root of the corresponding diagonal element of the variance–covariance matrix C , that is, the error of β j is √ C jj . As shown in the top panel in Fig. 3b , the fit gives Γ 10 =34.2±0.7 GHz. The same algorithm is used to retrieve other relaxation rates and the corresponding errors listed in Tables 1 and 3 . Measurement of dipole moments This section describes how the dipole moments are extracted from the 3DFT spectrum along with the power measurements of the excitation laser beams and the FWM signal beam. Starting from the optical Bloch equations and assuming the pulse duration is much shorter than any dynamics or detunings, the FWM third-order polarization associated with peak 3A in the 3DFT spectrum in Fig. 2 is where N is the atomic density, E A,B,C are the electric field amplitudes of the excitation pulses, Γ 10 and Γ 21 are the dephasing rates, and the Θ’s are unit step functions. The factor of 2 is due to the two quantum pathways in peak 3A. For the sake of simplicity, the time delays τ and T can be set to zero for the power measurement of the FWM signal. Therefore, the polarization is The FWM polarization of all other 3DFT peaks in Fig. 2 can be written in a similar form except for different dipole moments. Since the D 1 and D 2 transitions have similar dephasing rates ( Γ 10 ≈ Γ 20 ), the FWM signal strength of each peak depends on the dipole moments as Designating the ratio of μ 02 to μ 01 as λ , that is, μ 02 = λμ 01 , the summation of all terms gives where is given by equation (9). The far-field electric field radiated by the polarization is where l is the sample length, n is the index of refraction, c is the speed of light in vacuum, is the vacuum permittivity and ω is the angular frequency of the emission. The intensity of the signal is This is the FWM signal intensity of a single shot. Therefore, the average power of the generated FWM signal is where A is the area of the laser beam cross section and f rep is the laser repetition rate. In equation (19), all parameters can be measured experimentally in order to calculate the dipole moments. Besides the parameters that can be easily measured, the atomic density N is determined by the temperature of the molten potassium held in the side arm of the vapour cell through the equation of state [45] , the dephasing rates are extracted from the lineshape analysis of 3DFT spectrum, and the electric field strength is derived from the measured laser power and the beam size at the sample position. The more challenging part is how to determine the ratio λ from the 3DFT spectrum and how to measure the average power of the FWM signal, which are described in the following. The relative strength of dipole moments μ 01 and μ 02 can be determined by comparing the peak amplitudes of peaks 3A and 3B and the laser spectral intensities at the corresponding frequencies. Specifically, the peak amplitudes of peaks 3A and 3B are where S 0,3A ( S 0,3A ) is the peak amplitude of peak 3A (3B), and I 01 ( I 02 ) is the laser spectral intensity at the frequency of D 1 ( D 2 ) transition. Therefore, the ratio is From the 3DFT spectrum in Fig. 2 , we measured S 0,3A =136±2.7 and S 0,3B =133±2.7. The laser intensities at the corresponding frequencies are I 01 =9,685±99 counts and I 02 =4,042±64 counts. Plug them into equation (22), we obtain the ratio λ =1.38±0.04. To measure the power of FWM signal in our experiment, the challenge is that the FWM signal is too weak to be measured by a conventional power meter. A photodiode and a lock-in amplifier are used to measure the time-integrated FWM signal. In order to measure the power of the signal, we first need to calibrate the detection system with the tracer beam whose power is high enough to be measured by a power meter. With the box geometry in the set-up shown in Fig. 6, the tracer beam propagates in the same direction as the FWM signal. In the calibration process, beams A, B and C are blocked while the tracer beam goes through the sample and is chopped for the lock-in detection. The photodiode is placed to optimize the signal from the tracer beam. Well-calibrated neutral density filters are inserted in the path such that both photodiode and lock-in amplifier are not saturated. The reading on the lock-in amplifier can then be calibrated to the actual power of the tracer beam measured by a power meter that is placed before the neutral density filters, and a conversion factor is obtained. Now we block the tracer beam and unblock beams A, B and C. The generated FWM signal is detected by the photodiode. Beam B is chopped for the lock-in detection. The reading on the lock-in amplifier includes the FWM signal and the background signal induced by beam B. This background can be measured with only beam B on and is subtracted to obtain the FWM signal. Using the conversion factor obtained in the calibration, the power of the FWM signal can be calculated from the lock-in amplifier reading. In our experiment, the measured FWM signal power is 2.38±0.24 nW, with the excitation power of 3.16±0.32 mW per beam. We note that the propagation effect is negligible, as the absorbance is smaller than 1 in our experiment, and the losses on the cell windows are calibrated when the cell is at the room temperature. The Gaussian distribution of the beam profile is considered in the calculation of field intensity. To estimate the uncertainty in the measurement of dipole moments, we have taken into account the uncertainties in all measured parameters. These include the uncertainties in the laser power (±10%), the FWM power (±10%), the cell temperature (±10 °C), the beam diameter (±10%), the pulse duration (±10%) and the sample length (±50%). In summary, using the measured parameters (with uncertainties) and equation (19), we obtained the dipole moments μ 01 =(1.8±0.83) × 10 −29 C m and μ 02 = λ (1.8±0.83) × 10 −29 C m, where the relative strength λ =1.38±0.04. How to cite this article: Li, H. et al. Unraveling quantum pathways using optical 3D Fourier-transform spectroscopy. Nat. Commun. 4:1390 doi: 10.1038/ncomms2405 (2013).